Palaeoclimate reconstructions reveal a strong link between El Niño-Southern Oscillation and Tropical Pacific mean state The El Niño-Southern Oscillation (ENSO) is one of the most important components of the global climate system, but its potential response to an anthropogenic increase in atmospheric CO 2 remains largely unknown. One of the major limitations in ENSO prediction is our poor understanding of the relationship between ENSO variability and long-term changes in Tropical Pacific oceanography. Here we investigate this relationship using palaeorecords derived from the geochemistry of planktonic foraminifera. Our results indicate a strong negative correlation between ENSO variability and zonal gradient of sea-surface temperatures across the Tropical Pacific during the last 22 ky. This strong correlation implies a mechanistic link that tightly couples zonal sea-surface temperature gradient and ENSO variability during large climate changes and provides a unique insight into potential ENSO evolution in the future by suggesting enhanced ENSO variability under a global warming scenario. The El Niño-Southern Oscillation (ENSO) is the second largest source of climate variability after the solar cycle [1] . Its 2–7-year oscillations between positive (El Niño) and negative (La Niña) phases cause significant redistribution of heat and moisture fluxes across the planet with dramatic social and economic impacts [1] . The impacts of ENSO, and in particular of strong El Niño events, are wide-ranging and can be devastating for societies and ecosystems, including, for example, changed incidence of disease, reduced agricultural yields, droughts and floods, changed incidence of tropical cyclones, fishery collapse and forest fires [2] . As a result, the last few decades have seen a growing concern about how the climate system will respond to global warming. Current climate modelling experiments are equivocal in predicting future ENSO behaviour, being strongly model-dependent [3] , [4] . One of the major uncertainties that limits progress in the field of ENSO prediction is a relatively poor understanding of how changes in the Tropical Pacific mean state (long-term average distribution of oceanographic and atmosphere parameters across the Equatorial Pacific) affect the frequency and intensity of ENSO events (that is, ENSO variability) [4] . Climate palaeoreconstructions have the potential to provide important insights into how ENSO variability relates to the Tropical Pacific mean state. For example, climate underwent dramatic changes during the last 25 ky as the Earth’s climate changed from cold glacial to modern-day warm interglacial conditions. These large changes in climate boundary conditions affected the ENSO system and offer an opportunity to better understand the relationship between the Tropical Pacific mean state and ENSO variability [5] , [6] . In this work, we investigate the relationship between ENSO variability and the Tropical Pacific mean state using palaeorecords spanning the last 22 ky. Our results indicate a strong negative correlation between ENSO variability and zonal gradient of sea-surface temperatures (SSTs) across the Tropical Pacific. This strong correlation implies a mechanistic link that tightly couples these two parameters during large climate transitions and provides a unique insight into potential ENSO evolution in the future. A new palaeoceanographic record from the Equatorial Pacific A direct record of ENSO variability has been generated for the last 22 ky by reconstructing changes in temperature variations of subsurface waters near the Galapagos Islands, which lie at the heart of ENSO activity. We used several geochemical proxies based on foraminiferal shells extracted from sediment Core CD38-17P (01.36′04S; 90 25′32W, 2580, m) ( Fig. 1 ). Temperature variability was reconstructed for six key intervals (Modern: 1.6 ky; Early Holocene: 9.1 ky; Deglaciation: 12.5, 15.1 and 17.9 ky and the Last Glacial Maximum (LGM)—20.7 ky) using a novel approach that involves repetitive Mg/Ca, δ 18 O and δ 13 C analyses of small volume samples each comprising two shells of Neogloboquadrina dutertrei . N. dutertrei , a planktonic foraminifera, is an ideal proxy for reconstructing past ENSO behaviour as it inhabits subsurface waters (50–100 m) where temperature anomalies are largest during ENSO events and contribution of the seasonal cycle is minimal [7] . ( Supplementary Note 1 ). We also generated conventional down-core records of surface and subsurface temperatures using bulk Mg/Ca analyses of Globigerinoides ruber and N. dutertrei shells covering the past 22 ky. These temperature records represent multi-centennial averages of oceanographic conditions and were used to reconstruct zonal and meridional gradients of SSTs across the Equatorial Pacific by comparing them with existing Mg/Ca records (Methods, Supplementary Note 2 ). Zonal and meridional SST gradients are major parameters of ENSO mean state and, to a large extent, control the intensity of the Walker and Hadley circulations and ocean–atmospheric coupling in the Tropical Pacific [1] . 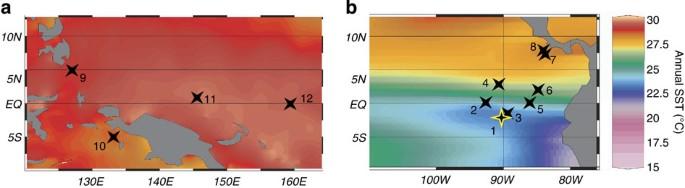Figure 1: Map of study area. Location map of sediment cores from the western equatorial Pacific (a) and eastern equatorial Pacific (b) used in reconstructing past oceanography of the Tropical Pacific. Stable warm-water conditions throughout the year characterize the eastern region, whereas the western side is typified by a strong seasonal cycle and upwelling of cold water off the coast of South America and the Galapagos Islands43. The seawater temperature gradient between these regions is one of the major driving forces of ENSO. Numbers on the map correspond to: 1—core CD38-17P, this study; 2—core TR163-22 (ref.44); 3—core VM21-30 (ref.45); 4—core TR163-19 (ref.46); 5—core ODP1240 (ref.47); 6—core ME-24JC48; 7—core ODP1242 (ref.42); 8—core MD02-2529 (ref.7); 9—MD98-2181 (ref.49); 10—core MD98-2176 (ref.49); 11—core MD97-2138 (ref.50); 12—core ODP 806 (ref.46); 13—core MD97-2141 (ref.51). Coloured background is modern-day annual mean sea-surface temperature from the World Ocean Atlas, 2001 (ref.43). Figure 1: Map of study area. Location map of sediment cores from the western equatorial Pacific ( a ) and eastern equatorial Pacific ( b ) used in reconstructing past oceanography of the Tropical Pacific. Stable warm-water conditions throughout the year characterize the eastern region, whereas the western side is typified by a strong seasonal cycle and upwelling of cold water off the coast of South America and the Galapagos Islands [43] . The seawater temperature gradient between these regions is one of the major driving forces of ENSO. Numbers on the map correspond to: 1—core CD38-17P, this study; 2—core TR163-22 (ref. 44 ); 3—core VM21-30 (ref. 45 ); 4—core TR163-19 (ref. 46 ); 5—core ODP1240 (ref. 47 ); 6—core ME-24JC [48] ; 7—core ODP1242 (ref. 42 ); 8—core MD02-2529 (ref. 7 ); 9—MD98-2181 (ref. 49 ); 10—core MD98-2176 (ref. 49 ); 11—core MD97-2138 (ref. 50 ); 12—core ODP 806 (ref. 46 ); 13—core MD97-2141 (ref. 51 ). Coloured background is modern-day annual mean sea-surface temperature from the World Ocean Atlas, 2001 (ref. 43 ). Full size image Changes in past ENSO variability The G. ruber Mg/Ca record of core CD38-17P shows that SSTs in the Galapagos region started to rise at around 17.5 ky, mimicking the ‘Antarctic’ deglaciation that is characterized by a gradual warming at 16–18 ky and a distinct minimum at 13 ky, which coincided with the Antarctic cold reversal ( Fig. 2a ). The variability of both Mg/Ca and δ 18 O values obtained using repetitive analyses of small volume samples of N. dutertrei ( Figs 2b,c and 3a–c ) show similar changes across the deglaciation. Minimal variability is recorded in the interval representing the early Holocene (9.1 ky), whereas largest variability is found during intervals corresponding to the glacial–interglacial transition (12.5, 15.1 and 17.9 ky) ( Fig. 3a–c ). The variability of Mg/Ca and δ 18 O values during the LGM interval are only slightly higher than those recorded for the late Holocene (for example, s.d. values of 0.40 vs 0.33 for Mg/Ca and 0.34 vs 0.28 for δ 18 O values, accordingly). 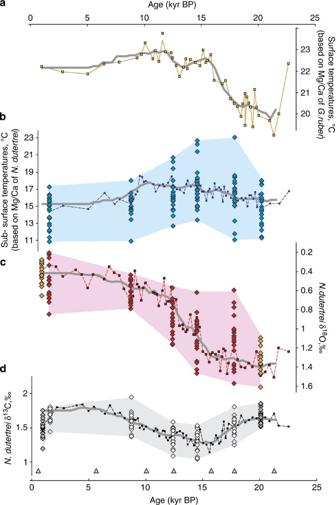Figure 2: Palaeoceanography of the Eastern Equatorial Pacific during the last 22 ky. (a) Changes in SST based on the Mg/Ca composition ofG. ruber(orange line and yellow squares) using thermometer calibration from Anandet al.40(b) Temperatures of subsurface waters based on the Mg/Ca composition ofN. dutertrei(blue squares) using thermometer calibration from Anandet al.40Blue diamonds represent temperature variability of subsurface waters calculated from repetitive Mg/Ca measurements ofN. dutertreisamples, each comprising two shells. Spread of these Mg/Ca values is shaded by light blue background. (c)N. dutertreiδ18O down-core record (red squares) and δ18O variability based on repetitive measurements ofN. dutertreisamples, each comprising two (red diamonds) to three shells (orange diamonds). Spread of these δ18O values is shaded by a pink red background. (d)N. dutertreiδ13C down-core record (black squares) and δ13C variability based on repetitive measurements ofN. dutertreisamples, each comprising two (white diamonds) to three shells (grey diamonds). Spread of these δ13C values is shaded by a light grey background. Grey triangles mark samples used for AMS14C dating. Thick grey lines denote 410 years running average extrapolated for each record. Figure 2: Palaeoceanography of the Eastern Equatorial Pacific during the last 22 ky. ( a ) Changes in SST based on the Mg/Ca composition of G. ruber (orange line and yellow squares) using thermometer calibration from Anand et al . [40] ( b ) Temperatures of subsurface waters based on the Mg/Ca composition of N. dutertrei (blue squares) using thermometer calibration from Anand et al . [40] Blue diamonds represent temperature variability of subsurface waters calculated from repetitive Mg/Ca measurements of N. dutertrei samples, each comprising two shells. Spread of these Mg/Ca values is shaded by light blue background. ( c ) N. dutertrei δ 18 O down-core record (red squares) and δ 18 O variability based on repetitive measurements of N. dutertrei samples, each comprising two (red diamonds) to three shells (orange diamonds). Spread of these δ 18 O values is shaded by a pink red background. ( d ) N. dutertrei δ 13 C down-core record (black squares) and δ 13 C variability based on repetitive measurements of N. dutertrei samples, each comprising two (white diamonds) to three shells (grey diamonds). Spread of these δ 13 C values is shaded by a light grey background. Grey triangles mark samples used for AMS 14 C dating. Thick grey lines denote 410 years running average extrapolated for each record. 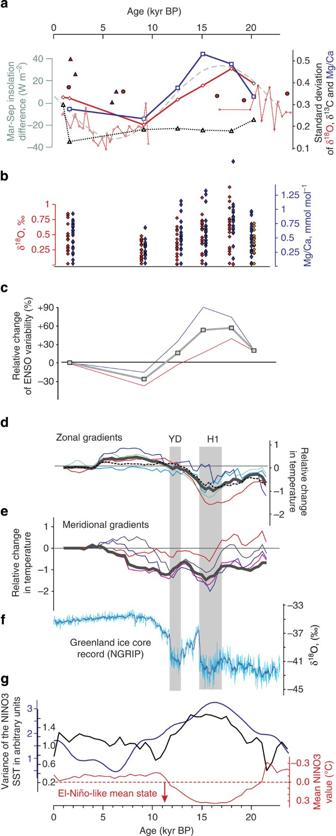Figure 3: ENSO variability and mean state during the last 22 ky. (a) s.d. of Mg/Ca (blue squares), δ18O (red diamonds) and δ13C (open black triangles) values from repetitive measurements ofN. dutertreitests (this study); δ18O ofG. ruber(closed purple triangles)45,52, (site 3,Fig. 1); δ18O ofN. dutertrei(closed red circles)7(site 8,Fig. 1);G. ruber(open red circles and dashed red line)15. Difference in solar insolation at equator in March and September representing amplitude of the seasonal cycle (dashed green line). (b) Range of Mg/Ca (blue) and δ18O (red) values recorded using repetitive analyses of small volume samples comprising two or three (LGM interval for δ18O values) shells ofN. dutertreinormalized to minimal values. (c) Relative change in ENSO variability expressed as % change from the earliest sample (1.5 ky). Changes in Mg/Ca (blue line) and δ18O (red line). Closed grey squares—average values for each time interval. (d) Changes in zonal gradient across the equatorial Pacific. Grey line—SST difference between the Eastern Pacific (average SST values from sites 1 and 7,Fig. 1) and the Western Pacific (average SST values from sites 9, 10, 11 and 12,Fig. 1). Thin lines—zonal gradient derived from subtracting our core SST values from sites 9 (green), 10 (red), 11 (dark blue) and 12 (light blue) inFig. 1. Black dashed line—zonal gradient calculated by subtracting average SST of all Eastern Equatorial Pacific (EEP) records from average SST of all Western Equatorial Pacific records. Grey blocks—Younger Dryas (YD) and Heinrich event (H1). (e) Changes in meridional gradient in the EEP. Grey line—SST difference between site 7 and sites 1 and 2,Fig. 1. Thin lines—zonal gradients calculated by subtracting our core SST from site 2 (red), site 5 (dark blue), site 4 (light blue), and site 7 (pink),Fig. 1. (f) Greenland ice core record53,54,55, grey line—running average. (g) Modelled changes in ENSO variability and mean state. Black line—change in ENSO variance. Red line—change in zonal gradient as per ref.13. Blue line—the change in ENSO variance as per Timmermannet al.56 Full size image Figure 3: ENSO variability and mean state during the last 22 ky. ( a ) s.d. of Mg/Ca (blue squares), δ 18 O (red diamonds) and δ 13 C (open black triangles) values from repetitive measurements of N. dutertrei tests (this study); δ 18 O of G. ruber (closed purple triangles) [45] , [52] , (site 3, Fig. 1 ); δ 18 O of N. dutertrei (closed red circles) [7] (site 8, Fig. 1 ); G. ruber (open red circles and dashed red line) [15] . Difference in solar insolation at equator in March and September representing amplitude of the seasonal cycle (dashed green line). ( b ) Range of Mg/Ca (blue) and δ 18 O (red) values recorded using repetitive analyses of small volume samples comprising two or three (LGM interval for δ 18 O values) shells of N. dutertrei normalized to minimal values. ( c ) Relative change in ENSO variability expressed as % change from the earliest sample (1.5 ky). Changes in Mg/Ca (blue line) and δ 18 O (red line). Closed grey squares—average values for each time interval. ( d ) Changes in zonal gradient across the equatorial Pacific. Grey line—SST difference between the Eastern Pacific (average SST values from sites 1 and 7, Fig. 1 ) and the Western Pacific (average SST values from sites 9, 10, 11 and 12, Fig. 1 ). Thin lines—zonal gradient derived from subtracting our core SST values from sites 9 (green), 10 (red), 11 (dark blue) and 12 (light blue) in Fig. 1 . Black dashed line—zonal gradient calculated by subtracting average SST of all Eastern Equatorial Pacific (EEP) records from average SST of all Western Equatorial Pacific records. Grey blocks—Younger Dryas (YD) and Heinrich event (H1). ( e ) Changes in meridional gradient in the EEP. Grey line—SST difference between site 7 and sites 1 and 2, Fig. 1 . Thin lines—zonal gradients calculated by subtracting our core SST from site 2 (red), site 5 (dark blue), site 4 (light blue), and site 7 (pink), Fig. 1 . ( f ) Greenland ice core record [53] , [54] , [55] , grey line—running average. ( g ) Modelled changes in ENSO variability and mean state. Black line—change in ENSO variance. Red line—change in zonal gradient as per ref. 13 . Blue line—the change in ENSO variance as per Timmermann et al . [56] Full size image Changes in ENSO variability were reconstructed using the s.d. values of both Mg/Ca and δ 18 O values converted into relative % change against modern-day ENSO variability that is recorded in the youngest core interval (1.6 ky) (Methods). ENSO variability was ∼ 20% higher than the modern-day during the LGM and increased significantly during early deglaciation (for example, 17.9 and at 15.1 ky interval). At 12.5 ky, ENSO variability is reduced to almost the modern-day value before further declining to ∼ 27% in the early Holocene (9.1 ky). Evolution of the Tropical Pacific mean state Changes in both zonal and meridional SST gradients are gradual and are within 1.5°C of modern-day values ( Fig. 3d–f ) ( Supplementary Discussion ). The zonal SST gradient was reduced throughout the LGM and during the early termination before reaching its minimal value at around 16–15.5 ky ( Fig. 3d ). The modern-day zonal gradient was established around the late deglaciation and was only slightly stronger during the Early and Middle Holocene ( Fig. 3d ). The meridional SST gradient, on the other hand, is reduced over most of the record and reached modern-day values only at around 4 ky ( Fig. 3e ). The meridional gradient also shows significant oscillations during the deglaciation, with minima centred at 16.5–14.5 and 10.5–11.5 ky intervals. It is worth noting that the pattern of changes in both gradients display strong similarities with Greenland Ice core δ 18 O records and therefore suggest a link between climate changes in the high-latitude Northern Hemisphere and the Tropical Pacific. This resemblance is particularly pronounced in changes in the meridional gradient of SST ( Fig. 3e,f ). Covariance of ENSO variance and Pacific oceanography The regression of our variability data against zonal and meridional SST gradients reveals an important link between ENSO variability and the Tropical Pacific mean state ( Fig. 4 ). There is a strong negative correlation ( R 2 =0.86; P =0.007) between variability of Mg/Ca values (that is, subsurface temperatures) and the zonal SST gradient ( Fig. 4 ). A similar correlation, but less statistically significant ( R 2 =0.78; P =0.02), is observed between variability of foraminiferal δ 18 O values and the zonal SST gradient. Our estimates of the relative change in ENSO variability (from Fig. 3c and derived from combining the aforementioned Mg/Ca and δ 18 O data) also have a strong and statistically significant negative correlation ( R 2 =0.94; P =0.002) with the zonal SST gradient. None of these relationships are observed for the meridional SST gradient. We estimate that 1% change in the zonal gradient corresponds to ∼ 3% change in ENSO variability. Recent studies of ENSO decadal variability during the late Holocene have indicated that intervals with increased ENSO variability usually coincided with decreased zonal SST gradients across the Pacific [8] , [9] . Our results suggest that this covariance is part of a larger-scale physical mechanism that tightly links ENSO variability and the zonal gradient across the Tropical Pacific and remains robust during at least the last 22 ky. The origin of this physical mechanism requires further investigation as none of the existing ENSO models can explicitly explain the observed relationship between ENSO variability and SST zonal gradient. Below we present a few possible hypotheses, which could offer some insights into the origin of this relationship. 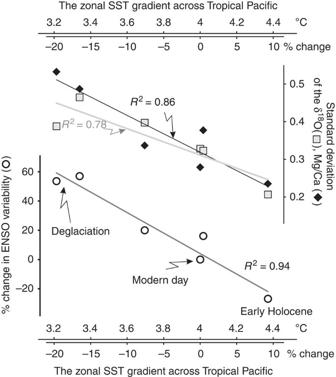Figure 4: Covariance between ENSO variability and Tropical Pacific mean state. ENSO variability is presented as: s.d. of Mg/Ca values ofN. dutertrei(black diamonds), s.d. of δ18O valuesN. dutertrei(white squares) and estimated % change in ENSO variability (open circles). The zonal gradient is calculated as the difference in SST between the Western Equatorial Pacific and the Eastern Equatorial Pacific (see Methods). All regressed parameters show significant correlation with the zonal gradient and underline the mechanism that links ENSO variability with the Tropical Pacific mean state during the last glacial–interglacial climate change. Figure 4: Covariance between ENSO variability and Tropical Pacific mean state. ENSO variability is presented as: s.d. of Mg/Ca values of N. dutertrei (black diamonds), s.d. of δ 18 O values N. dutertrei (white squares) and estimated % change in ENSO variability (open circles). The zonal gradient is calculated as the difference in SST between the Western Equatorial Pacific and the Eastern Equatorial Pacific (see Methods). All regressed parameters show significant correlation with the zonal gradient and underline the mechanism that links ENSO variability with the Tropical Pacific mean state during the last glacial–interglacial climate change. Full size image Climate modelling experiments have been used as a tool to help identify the factors that control ENSO variability, leading to a range of conclusions on the key drivers and processes. The classical ‘linear’ model links ENSO variability with the zonal gradient through the ‘destabilizing’ effect of cold thermocline waters of the Eastern Pacific but produced the opposite relationship [10] , [11] , [12] (for example, positive instead of negative correlation) compared with the results of our study. Another mechanism linking ENSO variability and SST zonal gradient is based on external forcing of one of several feedbacks within the ENSO system during a particular season [13] , [14] . Clement et al . [13] used this mechanism to demonstrate how orbital forcing, which is relatively weak in the tropics, could potentially modify the ENSO system at the precessional time scale. These modelling results show reasonable agreement with our data suggesting both increased (reduced) ENSO variability and reduced (increased) zonal gradients during the deglaciation (early Holocene) ( Fig. 3a,g ). Contrast between March and September solar insolation at the equator also closely follows the pattern of changes in ENSO variability [15] supporting the hypothesis by Clement et al . [13] However, recent complex coupled general circulation experiments [16] questioned these results. The intermediate complexity model (that is, the Cane and Zebiak model) used in the study by Clement et al . [13] requires prescribed, but poorly known, ENSO mean state and therefore could lead to potential modelling artefacts [16] . An alternative mechanism, which could link ENSO variability and the zonal SST gradient, was suggested by Timmermann [17] to explain the origin of ENSO decadal variability. Analysing ENSO data from observations and modelling experiments, he found 10–20-year cycles within the ENSO system, which can be described as alternating periods of enhanced ENSO variability and decreased zonal gradient with periods of subdued ENSO variability and increased zonal gradient. These decadal changes were attributed to the nonlinear dynamics of the ENSO system [12] , [18] , [19] . The nonlinear dynamic may be important for interpreting our results because the total variability reconstructed using proxy data represents a millennial average and consequently includes multiple components of ENSO variability. A close examination of other ENSO palaeorecords provides some support for this hypothesis. All sedimentary archives recording enhanced ENSO variability (for example, California margin, North America, New Zealand and Peru Margin) display strong multidecadal/centennial components [20] , [21] , [22] . Closest to our study site is a lithic-flux record off the Peru Margin, which shows that the 50–70-year frequency was dominant during intervals of increased ENSO variability, including the deglaciation interval analysed in this work. Considering this concurrence, we hypothesize that the strength of SST zonal gradient may have an important role in controlling the expression of the multidecadal/centennial component of ENSO variability. Accordingly, an increase in the amplitude of ENSO variability during periods such as the deglaciation evident in our record is reflecting enhanced decadal/centennial components of ENSO variability during these periods. A strong relationship between the zonal SST gradient and ENSO variability presents interesting implications for modern-day climate change and its effect on ENSO dynamics. The majority of the modelling experiments on future climate agree that increased greenhouse gases lead to weakening of the Walker circulation, which is usually accompanied by a decrease in the zonal SST gradient across the Equatorial Pacific [4] , [23] , [24] . If this is correct, then according to our findings, a reduced zonal gradient should enhance ENSO variability. Indeed, this is consistent with the observations that after 1970 the ENSO system was marked by two of the strongest El Niño events on record (the 1982/83 and 1997/98 events) and a prominent shift within ENSO feedbacks [25] , [26] . The exact mechanism of the post 1970 modification in the ENSO system is generally attributed to either global warming or decadal variability within ENSO [25] , [27] . In view of our results, both of these hypotheses could potentially reflect the same process of modification of the Walker circulation/ENSO mean state by global warming and its effect on ENSO variability, particularly on its multidecadal/centennial components. Geochemical analyses of sediment core material Piston core CD38-17p was collected in the Eastern Equatorial Pacific (EEP) (01.36′04S; 90 25′32W, 2580, m) during research cruise CD38′ in 1989 on the RRS ‘Charles Darwin’. The core was stored in the Edinburgh core repository and was only opened in 2009 preserving original undisturbed soft sediment. One half of the core was subsampled every centimetre for geochemical analyses of foraminifera and alkenones. Core sediment was freeze-dried and then washed using a 70-μm sieve to separate foraminiferal size fraction from clays. Geochemical analyses were done on two planktonic foraminifera; N. dutertrei and G. ruber . Three types of geochemical analyses were undertaken, conventional bulk measurements of Mg/Ca, δ 18 O, δ 13 C of N. dutertrei and G. ruber tests, which were later used for reconstructions of the ENSO mean state; repetitive analyses of the Mg/Ca, δ 18 O and δ 13 C but using small volume samples (2–3 tests) of N. dutertrei for study of past ENSO variability; and alkenone-derived U k 37 index. Bulk and repetitive Mg/Ca analyses Analyses were done at the University of Edinburgh using the inductively coupled plasma optical emission spectrometer (ICP-OES) facility. For the bulk measurement, we picked 40 tests of N. dutertrei from size fractions 400–450 μm and 35 tests of G. ruber from size fractions 250–350 μm. Repetitive analyses were done for six core intervals (Modern—1.6 ky; Early Holocene—9.1 ky; Deglaciation—12.5 ky, 15.1 ky, 17.9 ky and Last Glacial Maximum—20.7 ky). A total of 24 samples were analysed for each core interval comprising two tests of N. dutertrei in each sample. All samples were cleaned before geochemical analyses using a slightly modified version of the Barker et al . [28] method for trace-metal analyses in foraminifera. The modification includes use of an automatic cleaning system ( fOraccle , http://www.geminitechnologyltd.com ), which operates chemical steps of the cleaning protocol followed by substitution of the leaching step with weak nitric acid at the end of the cleaning protocol with a similar brief (2 min) rinsing step using 1 M ammonium citrate buffered with ammonia. Automation of the cleaning protocol provides greater cleaning efficiency as well as allowing cleaning small samples containing 1–2 foraminiferal tests, which is essential for this work. The Mg/Ca measurements were done using the standard protocol for Mg/Ca analyses of foraminiferal calcite [29] using Varian VISTA Pro ICP-OES. The long-term external precision of Mg/Ca analysis was monitored using ECRM 752-1 (ref. 30 ) and was about 0.02 mmol mol −1 (1 σ), which is equivalent of ∼ 0.5°C. Bulk δ 18 O and δ 13 C analyses Analyses on both N. dutertrei and G. ruber were done in the Stable Isotope Laboratory of University of Californa, Davis, using Micromass Optima isotope ratio mass spectrometer and standard lab protocol outlined in the study by Spero et al . [31] N. dutertrei samples comprised 15 tests picked from size fractions 400–450 μm, whereas G. ruber samples have 30 tests in each sample from size fractions 250–350 μm. Analytical precision was ±0.05% and ±0.04% for δ 18 O and δ 13 C, respectively, (±1 σ) based on repeat analyses of a NBS-19 calcite standard. Repetitive analyses of N. dutertrei δ 18 O and δ 13 C values Small volume repetitive analyses were done in Wolfson Laboratory, University of Edinburgh using a THERMO Electron Delta+ ADVANTAGE isotope ratio mass spectrometer. The analyses were done for seven core intervals (Core-top—0.7 ky, Modern—1.6 ky; Early Holocene—9.1 ky; Deglaciation—12.5 ky, 15.1 ky, 17.9 ky and the Last Glacial Maximum—20.7 ky). For the first and last intervals, we analysed 20 samples, each containing three tests of N. dutertrei . For the other core intervals and core-top interval, we analysed 20 samples but each sample from these intervals comprised two tests of N. dutertrei. This difference in shell numbers was designed to statistically characterize sample population and calculate the s.d. of each core interval. Typical analytical precision was ±0.09 and ±0.06% for δ 18 O and δ 13 C, respectively, (±1 σ) based on repeat analyses of the in-house standard. Alkenone analysis Alkenones were extracted from freeze-dried, homogenized aliquots of sediment using microwave-assisted extraction with dichloromethane and methanol (3:1, v-v;) [32] . Known concentrations of n-tetracontane (>98%, Sigma 87096) were added as an internal standard. An aliquot of the lipid extract was derivatized using bis(trimethylsilyl)trifluoroacetamide (Sigma Aldrich) by heating to 70°C for 1 h and then leaving overnight. The derivatized extract was analysed using a gas chromatograph fitted with a flame ionization detector to determine alkenone concentrations and the UK′37 index. Separation was achieved using an HP-1MS gas chromatography column (fused silica capillary column, 30 m × 0.25 mm i.d., coated with a 0.25 μm dimethyl polysiloxane phase). Helium was used as the carrier gas, and the oven temperature was programmed as follows: 60–200 °C at 20 °C min −1 , 200–320 °C at 6 °C min −1 , held at 310 °C for 35 min. Alkenone concentrations were calculated with reference to the internal standard (n-tetracontane). The relative concentrations of the di- and tri-unsaturated C37 alkenones were used to calculate the UK′37 index according to Prahl and Wakeham [33] : SSTs were calculated using the global mean annual sea-surface (0 m water depth) temperature calibration of Müller et al . [34] : Replicate extraction and analysis of selected samples determined that the average analytical reproducibility of this procedure is ±0.6 °C. Age model The core age model is based on seven accelerator mass spectrometer (AMS) 14 C dates ( Fig. 2 and Supplementary Fig. S1 ). AMS measurements were done in the Natural Environment Research Council radiocarbon facility at SUERC in East Kilbride. The program Calib6 (ref. 35 ) was used for calibration ( Supplementary Fig. S1a ). We used polynomial fit through calibrated ages to extrapolate the age model for the core interval of 0–25 ky. Estimating errors of the age model was carried out using Clam [36] and Bacon [37] methods. Both models agree well with our polynomial fit ( Supplementary Fig. S1b,c ). We also estimated errors for each interval studied for ENSO variability. The largest error was found for the Middle Holocene ( ∼ ±1,000 years), whereas the youngest deglaciation interval (that is, 12.5 ky) had the smallest error (±500 years). Considering that sediment bioturbation is usually 5–10 cm (ref. 38 ) or ∼ 750–1,500 years it is clear that age model errors are not the primary factor controlling uncertainty of the age estimation. Calculations of ENSO variability and ENSO mean state Calculations were based on the geochemistry of N. duterteri from the EEP. We used the s.d. from repetitive Mg/Ca and δ 18 O analyses as a measure for changes in ENSO variability across the deglaciation. Several considerations have been taken into account before converting our s.d. values into relative % change of ENSO variability. Measured s.d. values combined environmental variability recorded in the foraminiferal calcite and also variability of the analytical instrument (for example, ICP-OES or isotope ratio mass spectrometer (IRMS)) during each day of analyses. To subtract this instrumental variability, we analysed a reference standard every fifth sample and then subtracted variability recorded by this reference standard from total variability of each sample batch. Because both ICP-OES and IRMS were relatively stable throughout the analyses, analytical variability was only 2–5% of total variability for Mg/Ca measurements and 5–10% of total variability for δ 18 O measurements. The repetitive analyses of Mg/Ca and δ 18 O values were done using samples comprising two foraminiferal shells. Because we used two shells (and not one shell) our approach averaged some of the variability recorded by each proxy. To remove this averaging effect and also be able to directly compare our results with previously published work, which employed repetitive δ 18 O analyses on individual foraminiferal shells, we converted our s.d. into a new s.d., which assumed we measured each individual shell. This recalculation is done using the basic statistical principal of normal distribution where s.d. is a function from number of shells per sample ( Supplementary Fig. S2 ). To confirm that this normal distribution is applicable to our work, we analysed one of the core intervals twice using a similar repetitive approach but with a different number of shells per sample. One set of samples was prepared using two shells per sample and the other set using three shells per sample. Calculated s.d. values from both sets were later compared with predicted s.d. values by statistics. Measured and predicted values agreed well, supporting the use of this method. The first work on variability of Mg/Ca values in foraminiferal population demonstrated that s.d. values of Mg/Ca values are strongly dependent on the amplitude of seasonal changes and potentially can be used as a proxy for palaeoseasonality. However, Sadekov et al . [39] also revealed that part of this variability is due to not only changes in the temperature of seawaters but also to the biological activity of foraminifera. This biological contribution was assumed to be constant for total population and related to the variability of Mg/Ca values across individual foraminiferal chambers. Because a proportion of this biological variability is unknown for N. dutertrei , it is impossible to convert measured s.d. values directly into absolute temperature variability in the studied area. Therefore, we used relative % change in s.d. values as a measure for change in ENSO variability. We used the youngest interval of the core (1.4 ky) as a reference point to which the remaining five intervals were normalized ( Fig. 3c ). To calculate total relative % change in ENSO variability for each interval, we used the average from the estimate of this change by each proxy (for example, Mg/Ca and δ 18 O variability). Please note that because s.d. for each core interval also includes constant contribution of biological variability it may underestimate real relative % change in ENSO variability for the core interval. Also, please note that different methods of calculations (for example, with or without biological variability) do not affect results of regression between the ENSO variability and ENSO zonal/meridional gradients reported in the manuscript because they assumed constant biological offset and therefore change data proportionally to the original values. Zonal and meridional gradients Gradients were calculated using SST palaeorecords from the Equatorial Pacific, which are based only on Mg/Ca of G. ruber . This selectivity was essential to minimize potential error in the gradient calculation, which could be associated with the use of different proxies or different proxy carriers . G. ruber is also the most commonly used species for palaeocenography of low latitudes and also one of the most studied species of planktonic foraminifera with the largest number of publications about its ecology, biology and distribution. Before calculating each gradient, we standardized all available palaeorecord-based G. ruber Mg/Ca values. Original Mg/Ca values we obtained for each record and we calculated SST for each data set using the thermometer of Anand et al . [40] Mg/Ca values of the records that employed reductive cleaning protocol during sample preparation were also corrected by a 15% decrease in Mg/Ca due to foraminiferal dissolution reported by Barker et al . [28] and Yu et al . [41] A summary of all SST records used for the Equatorial Pacific is presented in Supplementary Fig. S3 and shows reasonable consistency between these records. We used the SigmaPlot software to calculate the running average mean record extrapolated for each 410-year interval. These average records for each site were used later for all gradient calculations. The meridional gradient for the EEP was calculated using only two records. The first record is from the Galapagos region (core CD38-17 this work) where SST values are coldest (low-end member) and the second record is from the Panama Margin (core 1242, Benway et al . [42] ) where SST are maximal (high-end member). The other records from the EEP were not used to avoid potential bias in the gradient calculation due to the relative contribution of each core resulting from the influence of the strong meridionally oriented oceanographic front just north of the Galapagos Islands. The zonal gradient was calculated by subtracting the average of the records from the Galapagos region (core CD38-17 this work) and the Panama Margin (core 1242, Benway et al . [42] ) from the average of the all available records from the Western Equatorial Pacific (WEP). Again the other records from the EEP were not used due to potential errors in gradient calculation due to the oceanographic front. We also used different combinations of all cores for calculation of both gradients and found that selection of the cores does not significantly affect the pattern of changes in the gradients. This is primarily due to a reasonable agreement between the cores for each region (for example, the EEP or the WEP). How to cite this article: Sadekov, A. Y. et al . Palaeoclimate reconstructions reveal a strong link between El Niño-Southern Oscillation and Tropical Pacific mean state. Nat. Commun. 4:2692 doi: 10.1038/ncomms3692 (2013).